TheEscherichia coliTus–Terreplication fork barrier causes site-specific DNA replication perturbation in yeast Replication fork (RF) pausing occurs at both ‘programmed’ sites and non-physiological barriers (for example, DNA adducts). Programmed RF pausing is required for site-specific DNA replication termination in Escherichia coli , and this process requires the binding of the polar terminator protein, Tus, to specific DNA sequences called Ter . Here, we demonstrate that Tus –Ter modules also induce polar RF pausing when engineered into the Saccharomyces cerevisiae genome. This heterologous RF barrier is distinct from a number of previously characterized, protein-mediated, RF pause sites in yeast, as it is neither Tof1-dependent nor counteracted by the Rrm3 helicase. Although the yeast replisome can overcome RF pausing at Tus– Ter modules, this event triggers site-specific homologous recombination that requires the RecQ helicase, Sgs1, for its timely resolution. We propose that Tus– Ter can be utilized as a versatile, site-specific, heterologous DNA replication-perturbing system, with a variety of potential applications. Inhibition of DNA replication fork (RF) progression is a major threat to genome stability during the S-phase. Factors that can cause RF pausing include DNA-bound proteins, ongoing transcription, secondary structures in DNA and various types of DNA damage. Each of these factors has the potential to create persistently stalled RFs or other types of unresolved DNA structures (for example, regressed/collapsed RFs, or aberrant recombination intermediates) arising as a consequence of the processing of these obstacles [1] . These events can ultimately lead to genomic and/or epigenetic alterations. Precisely how cells respond to DNA replication perturbation depends on a combination of how, and at which genomic location, the RF becomes arrested. Although many proteins implicated in dealing with DNA replication stress have been described, our knowledge of precisely how these proteins are deployed is quite rudimentary. Indeed, analysis of site-specific DNA replication perturbation is a technically difficult issue to address because the use of DNA-damaging agents to stall RFs leads to multiple types of DNA lesions scattered throughout the genome at sites that cannot be controlled or predicted. Furthermore, DNA-damaging agents may create a variety of lesions that disrupt RF progression in different ways. Therefore, novel technologies to site-specifically disrupt DNA replication are required to permit detailed molecular analyses of stalled RFs and aid our understanding of how cells maintain genome stability during the S-phase. Interestingly, some protein-mediated RF pauses are ‘programmed’ physiological events that are required to orchestrate DNA replication with other cellular processes. Two of the best examples of these in yeast are the Fob1-mediated RF pause in the rDNA array in S. cerevisiae [2] , and the RTS1 barrier at the mating type locus in S. pombe [3] . One shared feature of these programmed RF pauses is that they rely on the evolutionarily conserved intra-S-phase checkpoint mediator, Tof1 S.c. /Swi1 S.p . , to signal the presence of the RF barrier to the replisome and/or stabilize paused RFs [3] , [4] , [5] , [6] . Although these can be regarded as specialist RF-pausing systems, both of these have been transferred successfully to ectopic genomic loci (within the same organism) to analyse the consequences of unscheduled RF pausing [5] , [7] , [8] . Other examples of endogenously occurring, protein-mediated RF pause sites include centromeres, dormant replication origins and transfer RNA ( tRNA ) genes [9] , [10] . It remains to be determined whether these represent inevitable RF conflicts (for example, due to their complex nucleoprotein architecture), or whether these RF pauses are also exploited as physiological events to facilitate normal cell cycle progression. In support of the latter theory, RF pausing at diverse protein–DNA barriers also requires Tof1 signalling to the replisome in S. cerevisiae [11] . The Rrm3 helicase is required to counteract the RF pausing that occurs at tRNA genes, centromeres, inactive replication origins and Fob1-RFB [10] , [12] . In the absence of Rrm3, over 1,000 natural protein–DNA RF pauses throughout the genome become markedly enhanced, leading to increased RF breakage [10] , [13] . Consistent with RF pausing at protein–DNA complexes being a universal threat to genome stability, Escherichia coli also possesses accessory DNA helicases that act to clear protein–DNA barriers ahead of RFs [14] . Indeed, protein–DNA complexes are frequent sources of RF pausing in this organism [15] . Interestingly, E. coli also exhibits at least one example of programmed RF pausing, and this process is required to coordinate efficient DNA replication termination and chromosome segregation. This is achieved by the binding of the Tus terminator protein to a specific double-stranded DNA sequence called Ter [16] . Tus binds asymmetrically to Ter and presents either a ‘restrictive’ (blocking) or ‘permissive’ (non-blocking) face to the advancing replisome. Ter sites are arranged in the E. coli genome such that Tus binding to Ter creates a polar RF barrier that acts to ‘trap’ the two converging RFs in a defined DNA replication termination zone that is diametrically opposite to the DNA replication origin ( oriC ) in the E. coli genome [17] . Because Tus– Ter in E. coli comprises a robust, bipartite RF barrier that is not present in eukaryotes, we investigated whether this system could be reconstituted in the genome of S. cerevisiae . Owing to its ease of genetic analysis coupled with the established range of specialized techniques to analyse DNA replication, this organism has been used extensively to identify and characterize various proteins required for tolerating DNA replication stress. Here, we demonstrate that short arrays of Tus– Ter repeats can function as polar RF-pausing modules when engineered into the yeast genome. Interestingly, the replication machinery can overcome RF pausing at Tus– Ter modules without the requirement for either Rrm3 or homologous recombination repair (HRR) proteins. Nevertheless, these interruptions to replisome progression induce site-specific recombination. The yeast RecQ helicase, Sgs1, is required to resolve the ensuing recombination intermediates, and unprocessed DNA structures persist in sgs1 mutants following RF pausing at Tus– Ter modules. Therefore, we describe a novel system to engineer site-specific, DNA double-strand break-independent, sister chromatid recombination during the S-phase. We propose that Tus– Ter can be utilized as a novel heterologous system to investigate the consequences of non-physiological DNA replication perturbation at any desired genomic locus. Tus– Ter modules cause polar RF pausing in yeast The 21-bp TerB sequence was chosen for these analyses because the Tus– TerB interaction is well characterized [18] , and the TerB sequence has the strongest RF-pausing efficiency in E. coli [19] . We inserted three TerB sequences interspersed with two short spacer sequences adjacent to two well-characterized and early firing origins, ARS305 on chromosome III (ChrIII) and ARS607 on chromosome VI (ChrVI) ( Fig. 1 ). The close proximity of these Tus– Ter modules to both of these efficient origins means that rightward-moving RFs emanating from these origins will be the first forks to encounter Tus– Ter after travelling ~2 kb from ARS305 or ~4 kb from ARS607 , respectively. Importantly, in both scenarios, the adjacent downstream origin is >30 kb away, ensuring unidirectional collisions between rightward-moving RFs and Tus– Ter modules. We engineered yeast strains that harbour a Tus– Ter module in either the restrictive or permissive orientation adjacent to ARS305 , combined with its reciprocal orientation adjacent to ARS607 . This simultaneous analysis of two loci permits in vivo comparisons between different configurations of Tus– Ter modules on independent chromosomes, and controls for any possible locus-specific effects. Strains overexpressing Tus from a galactose-inducible promoter (to ensure full occupancy of all TerB sites) were synchronously released from the G1-arrest into the S-phase, and DNA replication intermediates were analysed at these loci by neutral-neutral two-dimentional (2D) gel electrophoresis ( Fig. 1a ). This technique permits the spatiotemporal detection of various types of DNA replication intermediates arising in a defined restriction fragment, including DNA replication origins (bubbles), RFs (Y-arcs) and X-shaped sister chromatid junctions (SCJs) [20] , [21] . SCJs are specialized DNA structures that arise at DNA replication origins and link sister chromatids via putative hemicatenane-like junctions [21] . After 35 min following G1-release, when the majority of cells were in early S-phase, RFs and SCJs that are indicative of normal origin firing [20] , [21] were detectable in both of the analysed restriction fragments adjacent to ARS305 and ARS607 ( Fig. 1b ). We observed that, when Tus– Ter modules were arranged in the restrictive orientation, a population of paused RFs was also detectable as a discrete ‘RF pause spot’ on the Y-arc ( Fig. 1b ). This RF pause spot was detectable in both the ChrIII and ChrVI restriction fragments, suggesting that the Tus– Ter modules can function equivalently when placed in different genomic locations. Importantly, the RF pause spot was not detectable at either genomic locus when Tus– Ter modules were arranged in the permissive orientation, or when Tus was not expressed ( Fig. 1b ; Supplementary Fig. 1 ). Alternative restriction digests also confirmed that the location of the RF pause spot on the Y-arc always corresponded to the predicted location of the 3x Ter module (see below). Taken together, these data indicate that Tus– Ter retains its ability to function as a bipartite, and intrinsically polar, RF-pausing system when reconstituted in the S. cerevisiae genome. 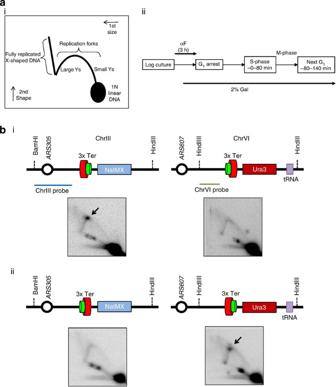Figure 1:E. coliTus–Terfunctions as a polar DNA replication fork barrier when reconstituted inS. cerevisiae. (a) (i) Diagram depicting the DNA replication intermediates that can be detected using neutral-neutral 2D gel electrophoresis of a defined restriction fragment. X-shaped DNA molecules may either comprise Rad51-independent sister chromatid junctions21or Rad51-dependent homologous recombination intermediates41. (ii) Schematic overview of the experimental procedure used to analyse RF pausing at Tus–Termodules. The approximate times for S- and M-phase progression are indicated. (b) Yeast strains were engineered with 3xTerBmodules adjacent toARS305(on ChrIII) andARS607(on ChrVI), such that these will be encountered in each case by rightward-moving DNA replication forks emanating from these origins in early S-phase. The 3xTerBmodules were arranged in either (i) the ChrIIIRESTRICTIVE/ChrVIPERMISSIVEorientation or (ii) the reciprocal ChrIIIPERMISSIVE/ChrVIRESTRICTIVEconfiguration. The diagrams depict the polarity of the 3xTerBmodules, and highlight the key features of interest at both chromosomal loci. Restriction enzyme sites are labelled, and the DNA replication origins are indicated as circles. The red section of Tus–TerB module represents the restrictive (blocking) face, whereas the green section represents the permissive (non-blocking) face. A natural tRNAApause site downstream of theTerBarray on ChrVI is also indicated as a purple box. Chromosome-specific probes are also indicated. The 2D gel images reveal DNA replication intermediates detectable at (BamHI-HindIII) ChrIII and (HindIII-HindIII) ChrVI restriction fragments following 35 min release from G1-arrest. Representative results are shown from a minimum of three independent experiments. A population of paused RFs at Tus–Teris indicated by the black arrow. Note that these stalled RFs are detectable only whenTerBsites are arranged in the restrictive configuration at each locus. Figure 1: E. coli Tus– Ter functions as a polar DNA replication fork barrier when reconstituted in S. cerevisiae . ( a ) (i) Diagram depicting the DNA replication intermediates that can be detected using neutral-neutral 2D gel electrophoresis of a defined restriction fragment. X-shaped DNA molecules may either comprise Rad51-independent sister chromatid junctions [21] or Rad51-dependent homologous recombination intermediates [41] . (ii) Schematic overview of the experimental procedure used to analyse RF pausing at Tus– Ter modules. The approximate times for S- and M-phase progression are indicated. ( b ) Yeast strains were engineered with 3x TerB modules adjacent to ARS305 (on ChrIII) and ARS607 (on ChrVI), such that these will be encountered in each case by rightward-moving DNA replication forks emanating from these origins in early S-phase. The 3x TerB modules were arranged in either (i) the ChrIII RESTRICTIVE /ChrVI PERMISSIVE orientation or (ii) the reciprocal ChrIII PERMISSIVE /ChrVI RESTRICTIVE configuration. The diagrams depict the polarity of the 3x TerB modules, and highlight the key features of interest at both chromosomal loci. Restriction enzyme sites are labelled, and the DNA replication origins are indicated as circles. The red section of Tus– Ter B module represents the restrictive (blocking) face, whereas the green section represents the permissive (non-blocking) face. A natural tRNA A pause site downstream of the TerB array on ChrVI is also indicated as a purple box. Chromosome-specific probes are also indicated. The 2D gel images reveal DNA replication intermediates detectable at (BamHI-HindIII) ChrIII and (HindIII-HindIII) ChrVI restriction fragments following 35 min release from G1-arrest. Representative results are shown from a minimum of three independent experiments. A population of paused RFs at Tus– Ter is indicated by the black arrow. Note that these stalled RFs are detectable only when TerB sites are arranged in the restrictive configuration at each locus. Full size image A critical role for a cytosine residue within TerB Two models have been proposed to explain how Tus– Ter functions as a polar RF barrier in E. coli . The ‘mousetrap’ model of Tus– Ter RF pausing posits that a specific interaction is required between Tus and a critical ‘locking cytosine’ residue within TerB that is revealed by DNA strand separation [22] . An alternative model proposes that RF arrest at Tus– Ter is mediated by specific protein–protein interactions in E. coli [23] , [24] . Our data suggest that, although additional proteins may be required to reinforce RF pausing at Tus– Ter in E. coli [23] , [24] , these are clearly not required for Tus– Ter to function as a polar RF barrier in yeast. We therefore investigated the consequences of mutating the putative ‘locking cytosine’ residue within the TerB sites inserted adjacent to ARS305 . We observed that a previously characterized C→T substitution [22] in each of the TerB sites adjacent to ARS305 abolished RF pausing ( Supplementary Fig. 2 ). Therefore, in agreement with Mulcair et al. [22] , this cytosine residue is critical for Tus– Ter to function as a polar RF barrier. This finding is somewhat surprising given the contrasting strand translocation polarities of the E. coli and yeast replicative helicases [25] . Indeed, the Tus– Ter barrier has specifically evolved to arrest the 5′ to 3′ DnaB helicase, and the cytosine capture event central to the mousetrap model should theoretically not be triggered by a 3′ to 5′ helicase (which would sequester the TerB critical cytosine within the central channel of the helicase and occlude its interaction with Tus) [22] . However, our demonstration that the cytosine residue in TerB is essential for Tus– Ter to arrest RFs in yeast suggests that strand separation may not necessarily always occur within the central channel of the MCM helicase in yeast. Tus– Ter modules cause transient RF pausing in yeast We observed that RF pausing at Tus– Ter modules was most pronounced at both origin-proximal restriction fragments analysed at ~35 min following G1-release ( Fig. 2 ). At this time, the ratio of stalled RFs to smaller (Y-shaped) RFs at the ChrIII and ChrVI triple Tus– Ter modules was 7.8 and 5.3, respectively ( Fig. 2 ). Comparable analyses conducted previously in E. coli demonstrated a ratio of 32.6 stalled:small RFs at a single, natural Tus– TerB locus [19] . This suggests that each individual Tus– TerB site is ~15-fold less efficient at holding RFs in yeast than in E. coli . However, as discussed below, this lower estimated efficiency in yeast probably also reflects the different outcomes following RF pausing in the respective organisms, as Tus– Ter functions as a stable RF-arresting complex in E. coli [26] , but can be overcome in yeast. Moreover, an important aspect of the system we developed is that we can increase the efficiency of RF pausing by increasing the number of TerB sites (see below). 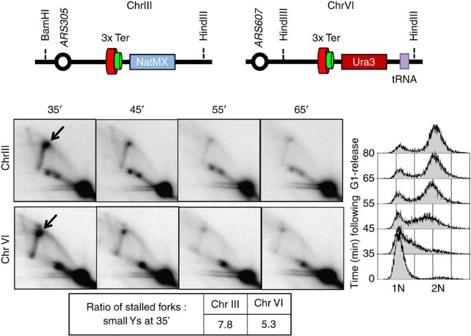Figure 2: The 3xTerBmodules cause transient replication fork pausing. A strain harbouring restrictive 3xTerBsites on both ChrIII and ChrVI (3xTerBChrIIIRESTRICTIVE/ChrVIRESTRICTIVE) was analysed. DNA replication intermediates adjacent toARS305(on ChrIII) andARS607(on ChrVI) were detected by 2D gel electrophoresis at the indicated times following G1-release, as described inFig. 1. Representative results are shown from a minimum of three independent experiments. RF pausing at Tus–Teris indicated by the black arrow. Flow cytometry data of cell cycle progression following release from G1-arrest (time 0) are also shown on the right. The ratio of stalled:small RFs was quantified at 35 min, and the values are shown underneath the 2D gel panel. Figure 2: The 3x TerB modules cause transient replication fork pausing. A strain harbouring restrictive 3x TerB sites on both ChrIII and ChrVI (3x TerB ChrIII RESTRICTIVE /ChrVI RESTRICTIVE ) was analysed. DNA replication intermediates adjacent to ARS305 (on ChrIII) and ARS607 (on ChrVI) were detected by 2D gel electrophoresis at the indicated times following G1-release, as described in Fig. 1 . Representative results are shown from a minimum of three independent experiments. RF pausing at Tus– Ter is indicated by the black arrow. Flow cytometry data of cell cycle progression following release from G1-arrest (time 0) are also shown on the right. The ratio of stalled:small RFs was quantified at 35 min, and the values are shown underneath the 2D gel panel. Full size image After ~35 min following G1-release, the intensity of the RF-pausing signal at the Tus– Ter modules began to diminish, and only a very small proportion of stalled RFs was detectable beyond 55 min ( Fig. 2 ). This decline in RF-pausing intensity correlated with the completion of bulk DNA replication and the disappearance of DNA replication intermediates on 2D gels. Increasing the number of Ter sites from three to seven could noticeably enhance the extent of RF pausing detectable at 35 min after G1-release, but this did not obviously affect cell viability or the kinetics of subsequent cell cycle progression ( Supplementary Fig. 1 ). Taken together, the data presented thus far indicate that Tus– Ter modules can induce polar RF pausing in yeast, but that yeast can tolerate these events. To investigate whether RF convergence was required to relieve RF pausing occurring at Tus– Ter modules, we inserted a second, tandem Tus– Ter module downstream of the restrictive 3x TerB module on ChrIII ( Supplementary Fig. 3A ). Because Tus– Ter modules retain their polarity and RF-arresting efficiency when placed in different genomic locations in yeast ( Figs 1 and 2 ), the second 3x TerB module was arranged in either the restrictive or permissive orientation to arrest either rightward- or leftward-moving RFs, respectively. We observed that the presence of a second permissive, ARS305 -distal, Tus– Ter module did not enhance the intensity, nor delay the resolution, of RF pausing at the origin-proximal Tus– Ter module ( Supplementary Fig. 3 ; ‘RES-per’ strain). This suggests that any leftward-moving RFs (that would have to travel ~34 kb from ARS306 ) are not required to relieve RF arrest at the origin-proximal Tus– Ter module. The second, ARS305 -distal, Tus– Ter module caused detectable RF pausing when arranged in the restrictive configuration ( Supplementary Fig. 3B ; ‘RES-RES’). In this scenario, the two tandem ‘RES-RES’ RF pauses diminished with similar kinetics to each other, and to the origin-proximal Tus– Ter module in the ‘RES-per’ strain ( Supplementary Fig. 3B ). We note that it was not possible to determine whether the two tandem RF pauses detectable in the ‘RES-RES’ strain were sequential transient RF pauses, or two independent RF pauses. Nevertheless, our data suggest that the S. cerevisiae replisome can overcome RF pausing at each Tus– Ter module, without the requirement for a convergence of two RFs. RF pausing at Tus– Ter modules is Tof1 and Rrm3 independent Tof1 S.c. /Swi1 S.p . is required to establish RF pausing at diverse types of endogenous RF pause sites in yeast [3] , [4] , [5] , [6] , [11] . Interestingly, however, we observed that RF pausing at Tus– Ter modules was detectable in tof1 mutants ( Supplementary Fig. 4 ). This indicates that the proposed role for Tof1 in establishing protein-mediated RF pauses is specific for certain types of endogenous protein–DNA pause sites. Because Rrm3 has been previously implicated as a ‘sweepase’ helicase that removes DNA-bound proteins that can impede DNA replication [10] , we investigated whether Rrm3 was required for RFs to overcome Tus– Ter modules. However, RF pausing at both of the ChrIII and ChrVI Tus– Ter modules was neither notably enhanced nor temporally extended, by deletion of RRM3 , despite the delay in bulk DNA replication completion occurring in this mutant ( Fig. 3 ). This characteristic DNA replication profile has been demonstrated previously for rrm3 mutants, and is proposed to be a consequence of increased origin usage, coupled with genome-wide RF stalling at >1,000 predicted sites in rrm3 mutants [10] , [27] , [28] , [29] . We also observed that two tandem arrays of 3x Ter modules (when the origin-distal array was arranged in either the permissive or restrictive orientation) behaved similarly in both wild-type and rrm3 strains ( Supplementary Fig. 3 ), suggesting that RF pausing and resumption at Tus– Ter modules occurred via similar mechanisms that were independent of Rrm3. Despite the apparent lack of contribution of Rrm3 to counteracting RF pausing at Tus– Ter modules, analysis of the Y-arc signal downstream of the Tus– Ter module on ChrVI confirmed the contribution of Rrm3 in overcoming a natural RF pause site occurring at the tRNA A (tA(AGC)F) gene [9] , [10] . We observed that this tRNA A pause site caused only minimal RF pausing in wild-type cells, but this was markedly enhanced in rrm3 mutants ( Fig. 3 ; Supplementary Fig. 5 ), demonstrating that Rrm3 is highly selective for counteracting this specific endogenous protein–DNA RF pause site. Taken together, our data demonstrate that RF pausing at Tus– Ter modules occurs independently of Tof1 or Rrm3, and is therefore mechanistically distinct from RF pausing that occurs at previously characterized, endogenous, protein-mediated RF pauses [10] , [11] . Hence, we propose that Tus– Ter is suitable for characterization of the cellular responses to an inadvertent encounter between a RF and a non-physiological obstruction. 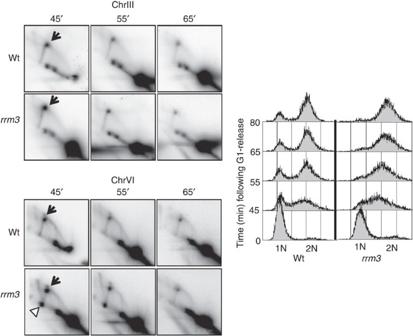Figure 3: Replication fork pausing at Tus–Termodules is not counteracted by the Rrm3 ‘sweepase’. The wild-type andrrm33xTerBChrIIIRESTRICTIVE/ChrVIRESTRICTIVEstrains were released from G1-arrest and DNA replication intermediates were detected by 2D gel electrophoresis at the indicated times. Representative results are shown from a minimum of three independent experiments. RF pausing at Tus–Teris indicated by the black arrow, and RF pausing at thetRNAAgene on ChrVI is indicated by the white arrowhead. Flow cytometry data are also shown. Figure 3: Replication fork pausing at Tus– Ter modules is not counteracted by the Rrm3 ‘sweepase’. The wild-type and rrm3 3x TerB ChrIII RESTRICTIVE /ChrVI RESTRICTIVE strains were released from G1-arrest and DNA replication intermediates were detected by 2D gel electrophoresis at the indicated times. Representative results are shown from a minimum of three independent experiments. RF pausing at Tus– Ter is indicated by the black arrow, and RF pausing at the tRNA A gene on ChrVI is indicated by the white arrowhead. Flow cytometry data are also shown. Full size image Mec1 signalling is not required to overcome RF pausing The DNA replication checkpoint is required to stabilize stalled RFs following DNA replication perturbation, and also promotes recovery from RF arrest [30] , [31] , [32] . However, we observed that RF pausing at Tus– Ter modules was not associated with any detectable activation of the checkpoint effector kinase, Rad53 ( Supplementary Fig. 1 ). To fully examine whether the S-phase checkpoint is required to overcome RF pausing at Tus– Ter modules, we investigated the consequences of deleting the central checkpoint kinase, Mec1, which acts upstream of Rad53 (refs 33 , 34 ). Because mec1 single mutants are inviable owing to Sml1-mediated inhibition of dNTP synthesis [35] , this was achieved by comparing the responses with Tus– Ter modules in sml1 versus sml1mec1 strains. Interestingly, however, we observed that RF pausing and resolution at Tus– Ter modules was indistinguishable in sml1 and sml1 mec1 mutants ( Fig. 4a ; Supplementary Fig. 6A ). This observation suggests that Mec1 signalling is not required to resume RF progression following RF pausing at Tus– Ter modules. 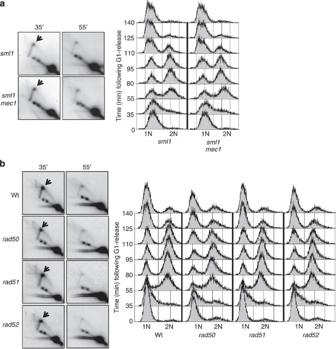Figure 4: Mec1-dependent checkpoint signalling and homologous recombination repair are not required to overcome replication fork pausing at Tus–Termodules. (a)sml1andsml1mec13xTerBChrIIIRESTRICTIVE/ChrVIRESTRICTIVEstrains were released from G1-arrest and DNA replication intermediates present at ChrIII were detected by 2D gels at the indicated times. Representative results are shown from a minimum of three independent experiments. RF pausing at Tus–Teris indicated by the black arrow. Flow cytometry data are also shown. The corresponding ChrVI data are shown inSupplementary Fig. 6. (b) Wild-type,rad50,rad51andrad523xTerBChrIIIRESTRICTIVE/ChrVIRESTRICTIVEstrains were analysed as described above. Figure 4: Mec1-dependent checkpoint signalling and homologous recombination repair are not required to overcome replication fork pausing at Tus– Ter modules. ( a ) sml1 and sml1mec1 3x TerB ChrIII RESTRICTIVE /ChrVI RESTRICTIVE strains were released from G1-arrest and DNA replication intermediates present at ChrIII were detected by 2D gels at the indicated times. Representative results are shown from a minimum of three independent experiments. RF pausing at Tus– Ter is indicated by the black arrow. Flow cytometry data are also shown. The corresponding ChrVI data are shown in Supplementary Fig. 6 . ( b ) Wild-type, rad50 , rad51 and rad52 3x TerB ChrIII RESTRICTIVE /ChrVI RESTRICTIVE strains were analysed as described above. Full size image Recombination is not required to overcome RF pausing HRR has been strongly implicated in the restart and repair of stalled RFs [36] . Indeed, the RTS1 RF barrier in S. pombe requires Rad22 (Rad52 S.c. ), Rad50 (Rad50 S.c. ) and Rhp51 (Rad51 S.c. ) for RF restart [8] , [37] . We therefore analysed the consequences of RF pausing at Tus– Ter modules in rad50 , rad51 and rad52 mutants. Interestingly, unlike the RTS1 barrier in S. pombe , we observed that deletion of each of these HRR proteins did not noticeably affect the extent or timing of RF pausing at Tus– Ter modules ( Fig. 4b ; Supplementary Fig. 6B ). In addition to suppressing genome instability at paused RFs, HRR is also required to repair any double-strand breaks (DSBs) arising at collapsed RFs by gene conversion, single-strand annealing or break-induced replication [38] . Indeed, a single DSB arising during the S-phase has been demonstrated to elicit a robust G2/M arrest in rad52 mutants [39] . However, we observed that mitotic progression occurred with wild-type-like kinetics following RF pausing at Tus– Ter in rad50 , rad51 or rad52 strains, suggesting that the G2/M checkpoint did not become activated ( Fig. 4b ). Taken together, our data suggest that HRR is not required to overcome Tus– Ter modules, and that RF collapse at Tus– Ter does not occur frequently in our system. RF pausing causes unprocessed DNA structures in sgs1 mutants Next, we analysed the contribution of the RecQ helicase, Sgs1 at stalled RFs. A number of putative roles have been proposed for RecQ helicases at perturbed RFs, including RF stabilization and RF restart [40] . We observed that Tus– Ter RF pausing and bypass kinetics, as well as subsequent mitotic progression and viability, were indistinguishable in sgs1 and wild-type cells ( Fig. 5a ; Supplementary Fig. 6C ). Interestingly, however, we observed that a fully replicated, X-shaped DNA structure was now detectable in sgs1 mutants ( Fig. 5a ; Supplementary Fig. 6C ). This X-structure was still detectable at 55 min, at which time SCJs (which comprise hemicatenane-like junctions formed at DNA replication origins [21] ) had disappeared. Furthermore, this X-structure (unlike SCJs) was Rad51 dependent, indicating that it comprised an unprocessed HRR intermediate ( Fig. 5a ; Supplementary Fig. 6C ). Importantly, the sgs1 X-structure was dependent on RF pausing at Tus– Ter , and did not arise when Ter sites were arranged in the permissive orientation ( Fig. 5b ). Furthermore, the signal intensity of the sgs1 X-structure was enhanced by increasing the number of Ter sites from three to seven ( Fig. 5b ), further demonstrating that this X-structure specifically arises as a consequence of RF pausing at Tus– Ter modules. Taken together, we propose that RF pausing at Tus– Ter modules elicits the formation of a Rad51-dependent HRR intermediate that is normally resolved by Sgs1. 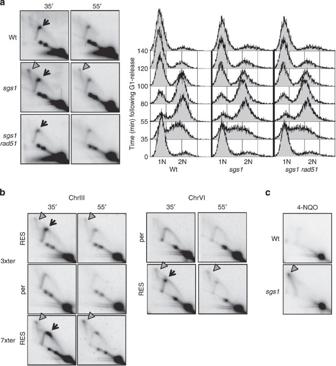Figure 5: Unprocessed X-structures persist insgs1mutants following RF pausing at Tus–Termodules. (a) Wild-type,sgs1andsgs1 rad513xTerBChrIIIRESTRICTIVE/ChrVIRESTRICTIVEstrains were released from G1-arrest, and DNA replication intermediates present at ChrIII were detected by 2D gels at the indicated times. Representative results are shown from a minimum of three independent experiments. RF pausing at Tus–Teris indicated by the black arrow. Flow cytometry data are also shown. Unprocessed X-shaped DNA molecules insgs1mutants are indicated by the grey arrowhead. Note the absence of this DNA structure in thesgs1 rad51double mutant. The corresponding ChrVI data are shown inSupplementary Fig. 6. (b)sgs1strains harbouring three different indicated configurations and numbers ofTermodules were analysed as described ina. Note that the 7xTerstrain does not contain anyTersites at ChrVI, and was therefore probed for ChrIII only. (c) Wild-type andsgs1strains (harbouringTersites, but not containing the Tus plasmid) were released from G1-arrest into medium containing 1 μg ml−14NQO. After 150 min, when cultures had traversed S-phase and were arrested in G2/M, DNA replication intermediates present at ChrIII were detected by 2D gels. Representative results are shown from a minimum of three independent experiments. Unprocessed X-shaped DNA molecules arising insgs1mutants are indicated by the grey arrowhead. Figure 5: Unprocessed X-structures persist in sgs1 mutants following RF pausing at Tus– Ter modules. ( a ) Wild-type, sgs1 and sgs1 rad51 3x TerB ChrIII RESTRICTIVE /ChrVI RESTRICTIVE strains were released from G1-arrest, and DNA replication intermediates present at ChrIII were detected by 2D gels at the indicated times. Representative results are shown from a minimum of three independent experiments. RF pausing at Tus– Ter is indicated by the black arrow. Flow cytometry data are also shown. Unprocessed X-shaped DNA molecules in sgs1 mutants are indicated by the grey arrowhead. Note the absence of this DNA structure in the sgs1 rad51 double mutant. The corresponding ChrVI data are shown in Supplementary Fig. 6 . ( b ) sgs1 strains harbouring three different indicated configurations and numbers of Ter modules were analysed as described in a . Note that the 7x Ter strain does not contain any Ter sites at ChrVI, and was therefore probed for ChrIII only. ( c ) Wild-type and sgs1 strains (harbouring Ter sites, but not containing the Tus plasmid) were released from G1-arrest into medium containing 1 μg ml −1 4NQO. After 150 min, when cultures had traversed S-phase and were arrested in G2/M, DNA replication intermediates present at ChrIII were detected by 2D gels. Representative results are shown from a minimum of three independent experiments. Unprocessed X-shaped DNA molecules arising in sgs1 mutants are indicated by the grey arrowhead. Full size image The sgs1 X-structure arising as a consequence of RF arrest at Tus– Ter modules is highly reminiscent of the post-replicative X-structures that persists in sgs1 mutants following exposure to the replication-perturbing agent, methylmethanesulphonate (MMS) [41] , [42] . This X-structure does not arise in hydroxyurea-treated sgs1 cells [41] , suggesting that it is not a general property of DNA replication stress, but rather arises in response to certain kinds of DNA replication impediments. To further examine whether unprocessed X-structures in sgs1 mutants are a general feature following disruption of DNA replication by non-physiological lesions or barriers, we compared the effects of exposing wild-type and sgs1 strains (harbouring TerB sites, but not expressing Tus) with 4-nitroquinoline 1-oxide (4NQO), which causes genome-wide bulky base adducts that mimic ultraviolet irradiation and cause RF stalling in yeast [43] . Interestingly, we observed that this agent, like MMS [41] and Tus– Ter modules, could also generate a post-replicative unprocessed X-structure in sgs1 mutants ( Fig. 5c ). We note, however, that despite being superficially similar to MMS-induced X-structures, the precise biophysical properties of the 4NQO-induced, or Tus– Ter -induced, X-structures await further detailed characterization. Nevertheless, our observations suggest that unprocessed X-structures arising in sgs1 mutants may be a general consequence following RF pausing at obstacles or lesions that impede DNA replication. The use of our Tus– Ter system will therefore permit these events occurring at stalled RFs, including the role(s) of Sgs1, to be analysed in a site-specific manner in future studies. To our knowledge, our reconstitution of bacterial Tus– Ter in yeast comprises the first heterologous, site-specific, protein-mediated, RF-pausing system characterized in a eukaryotic cell. The novelty of this system is reflected by the fact that, unlike all currently known endogenous RF pauses occurring throughout the S. cerevisiae genome, it does not require Tof1 for its establishment and is not counteracted by Rrm3 (refs 10 , 11 ). Rather, our data suggest that Tus– Ter modules form a site-specific RF barrier that superficially mimics either MMS or 4NQO lesions, and, consequently, induces site-specific recombination that requires the RecQ helicase, Sgs1, for its timely resolution. Interestingly, RF pausing at Tus– Ter modules can be overcome, suggesting that the yeast replisome is efficient at overcoming non-physiological DNA replication impediments. It will be of significant interest in future studies to determine the precise molecular events occurring at paused RFs at Tus– Ter modules. One interesting possibility is that the yeast replisome itself may physically destabilize (or actively trigger the localized degradation of) DNA-bound Tus following RF arrest. Importantly, because HRR is not required to restart RFs following pausing at Tus– Ter modules, our system can be distinguished from the RTS1 barrier previously characterized in S. pombe [8] , [37] . Rather, we propose that transient RF pausing at Tus– Ter modules may cause a site-specific single-stranded DNA (ssDNA) gap that is post-replicatively repaired by HRR. Indeed, in E. coli , the replisome can extend right up to Tus– Ter on the leading strand, and generates a ssDNA gap on the lagging strand [16] . Although RFs arrested at Tus– Ter are stable and not recombinogenic per se in E. coli [26] , we speculate that a similar process of ssDNA gap formation could have different consequences in yeast owing to the non-physiological nature of the RF pausing at Tus– Ter modules. Indeed, natural and non-physiological RF pauses are also processed differently in E. coli [26] . Taken together, our data indicate that the Tus– Ter system can be used to induce DSB-independent, site-specific, sister chromatid recombination during the S-phase. This novel methodology should circumvent the technically limited approach of using DNA-damaging agents (that elicit genome-wide DNA damage and loss of viability) to examine the consequences of DNA replication stress. In this respect, the use of Tus– Ter to study site-specific DNA replication perturbation is analogous to the use of the HO and I-SceI DNA nucleases that subsequently revolutionized the field of DNA DSB repair [38] , [44] , [45] . Although we have characterized physiological responses to RF stalling at Tus– Ter modules placed adjacent to efficient early replication origins in yeast, this system could also be used to (i) examine the cellular responses to RF stalling at other genomic loci, including late-replicating or intrinsically fragile regions, and (ii) analyse protein recruitment, post-translational modifications and DNA topological transitions occurring at each of these engineered RF pauses. Furthermore, because RF pausing at Tus– Ter modules can be augmented by the addition of more Ter sites, the Tus– Ter system could be specifically engineered to create transient or more robust RF pausing depending on the desired outcome. We propose therefore that Tus– Ter comprises a novel and versatile system that will permit the detailed analysis of the consequences of site-specific DNA replication perturbation in unprecedented detail. Unless indicated otherwise, all reagents were purchased from Sigma-Aldrich. Strains and plasmids The E. coli Tus gene was fused to a C-terminal NLS (PKKKRKV) during PCR amplification and cloned into the single copy p415-GAL1 ( ARS CEN LEU2 ) plasmid, to place Tus expression under the control of a galactose-inducible promoter [46] . All yeast strains used in this study are isogenic derivatives of BY4741. TerB modules, open-reading frame (ORF) deletion cassettes and yeast marker-swap cassettes were all integrated into the yeast genome by targeted homologous recombination [47] . The TerB modules (each containing short interspersed regions of random DNA sequences between each TerB sites) were constructed in vitro using synthetic oligonucleotides, and then cloned into YCplac33 or pBlu2SK plasmids so that they were adjacent to the yeast URA3 selectable marker. The 94-bp 3x TerB ‘restrictive’ module, as arranged on the Watson (5′→3′) strand in the yeast genome, consisted of the following sequence: 5′-ATAA G TATGTTGTAACTAAAGTTAAGCCTGTATTCGA ATAA G TATGTTGTAACTAAAG TTGACAGATCTTCAA ATAA G TATGTTGTAACTAAAG -3 ′. The 21-bp TerB -restrictive sequences (that have been previously validated by surface plasmid resonance [18] ) are indicated in bold font. The 94-bp 3x TerB ‘permissive’ module used in this study was antiparallel to the 3x TerB ‘restrictive’ module. The putative ‘locking cytosine’ residue (which is a guanine in this orientation) residue within TerB repeats is underlined. This residue was replaced with an adenine (A) residue in the 3x TerB ‘locking cytosine substitution’ module. The 7x TerB ‘restrictive’ module used in this study consisted of the following sequence: 5′- ATAA G TATGTTGTAACTAAAG TCCATGCAGGACGTCTTGGA ATAA G TATGTTGTAACTAAAG TTAAGCCTGTATTCGG ATAA G TATGTTGTAACTAAAG TTGACAGATCTTCAA ATAA G TATGTTGTAACTAAAG TCCATGCAGGACGTCTCGGA ATAA G TATGTTGTAACTAAAG TTAAGCCTGTATTCGA ATAA G TATGTTGTAACTAAAG TTGACAGATCTTCAA ATAA G TATGTTGTAACTAAAG -3 ′. The TerB modules (and a URA3 selectable marker) were then integrated into the yeast genome via the generation of PCR products with flanking targeting sequences. Two genomic locations were used in this study. The Chromosome III location was based on a previous study by Lopes et al. [48] , and the TerB modules were inserted between two non-essential ORFs ( YCL049C and YCL048W ), located ~2 kb to the right of ARS305 . The following 65-bp primer sequences were used as PCR-product overhangs to target TerB modules into the Chromosome III location: 5′-GAGCAAGACAAACAGGGCCAGCTGATGCATATGTTTTGTGTTGCTTTCCTACGATCAGCTAATGC-3′, and 5′-GGAAAATGAGTTTTGTCCCACCTTCCCTTTGGGAAAAGGCAATGTAAATCTTAGAGGCAAGAACC-3′. The Chromosome VI location was a complete gene replacement of the HIS2 ORF, located ~4 kb to the right of ARS607 . The following 65-bp primer sequences were used as PCR-product overhangs to target TerB modules into the Chromosome VI location: 5′-ACACAGCTGTACATGAGTTTATATGACAGTTTTTTTTTATGTACATCCAGTTCAAGATAATCAGA-3′, and 5′-CTTTCCCTTTCAAACACATTTTAGTACTTCTTGATACGTACAATTCAGTAAAAATCCTCGAGGTC-3′. Replacement of the URA3 marker with a NatMX cassette at the Chromosome III location was also achieved by targeted homologous recombination. To construct the ChrIII RES-RES or RES-PER module, a strain harbouring an origin-proximal 3x TerB - NatMX module was transformed with a HphMX -3x TerB cassette that was designed to replace the NatMX marker and create the 3x TerB - HphMX -3x TerB module. All Ter -harbouring yeast strains were verified by sequencing to ensure they contained the correct number and orientation of Ter sites in the genome. Full sequences are available on request. Yeast growth conditions and cell synchronization Yeast cultures were grown overnight in yeast extract peptone medium (Formedium, UK) supplemented with 3% sodium DL -lactate solution. Cultures were synchronized in G1 with alpha factor mating pheromone for 3 h (CASLO ApS, Denmark). Tus expression was induced by adding 2% Galactose (final w/v) for the final 2.5 h of the G1-arrest. Release of cells from G1-arrest was achieved by centrifugation, washing and resuspension of cells in fresh medium. After 1 h of G1-release (when cells were in late S-phase), alpha factor was added to the cultures to arrest cells in G1 after they have traversed the first mitosis, thus preventing a second round of DNA replication. For the analyses described in Fig. 5c , the indicated strains were released from G1-arrest into medium containing 4NQO at a final concentration of 1 μg ml −1 . Flow cytometry analysis One millilitre of cells were harvested by centrifugation and then fixed in 70% ethanol overnight. Cells were washed and resuspended in 1 ml of 50 mM sodium citrate (pH 7.0). Cells were briefly sonicated, and then treated with 0.25 mg ml −1 RNase A for 1 h at 50 °C. Proteinase K was then added to a final concentration of 1 mg ml −1 , and cells were incubated for a further 1 h at 50 °C. Samples were then diluted in 50 mM sodium citrate containing 16 μg ml −1 of propidium iodide, and incubated at room temperature for a minimum of 30 min. Samples were analysed using a Becton Dickinson FACSCalibur machine, using CellQuest software (BD Biosciences, Denmark). 2D gel analysis of DNA structures The hexadecyltrimethylammonium bromide (CTAB) method of DNA extraction was used [21] , [49] . An extensive version of this protocol has been described previously [49] . Briefly, 200 ml aliquots of cells were killed by the addition of 0.1% (final w/v) sodium azide at defined time points, and harvested by centrifugation. Spheroplasts were prepared by incubating cells in 5 ml of spheroplast buffer (1 M sorbitol, 100 mM EDTA pH 8.0, 0.1% β-mercaptoethanol, 100 U ml −1 zymolyase (AMSBIO, UK)) for 1 h at 30 °C. Following centrifugation, spheroplasts were then lysed in 2 ml water. To this, 2.5 ml of Solution I (2% w/v CTAB, 1.4 M NaCl, 100 mM Tris HCl pH 7.6, 25 mM EDTA pH 8.0) and 200 μl of 10 mg ml −1 RNase A were added, and samples were incubated at 50 °C. After 30 min, 200 μl of 20 mg ml −1 Proteinase K was added, and samples were incubated for a further 90 min at 50 °C. After this time, a further 100 μl of 20 mg ml −1 Proteinase K was added, and samples were incubated overnight at 30 °C. The next day, the supernatant (1) and pellet (2) were separated by centrifugation and treated as follows. (1) The supernatant was combined with 2.5 ml of 24:1 chloroform:isoamylalcohol, mixed and clarified by centrifugation. The upper phase was transferred to KIMBLE HS Borosilicate glass centrifuge tubes (Ettore Pasquali, Italy) containing 10 ml of Solution II (1% CTAB, 50 mM Tris HCl pH 7.6, 10 mM EDTA). After 1 h, the sample was centrifuged and the precipitate was resuspended in 2.5 ml of Solution III (1.4 M NaCl, 10 mM Tris HCl pH 7.6, 1 mM EDTA). (2) The pellet was resuspended in 2 ml of Solution III and incubated at 50 °C for 1 h. This was combined with 2.5 ml of 24:1 chloroform:isoamylalcohol, mixed and clarified by centrifugation. The upper phase was combined with the resuspended DNA from step (1). The DNA was then ethanol precipitated and resuspended in 10 mM Tris HCl pH 8.0. For each 2D gel image, 20 μg of DNA was digested overnight with the indicated restriction enzymes. The DNA was ethanol precipitated and resuspended in 20 μl of Tris-EDTA buffer. Samples were run on 0.35% low EEO agarose (US Biological, USA) first-dimensional gels at 50 V for ~21 h, and then stained with 0.3 μg ml −1 ethidium bromide. Gel strips were cut from first-dimensional gels and run on 0.90% agarose second-dimensional gels at 180 V (in Tris-borate-EDTA buffer containing 0.3 μg ml −1 ethidium bromide) for ~8 h. DNA was transferred to Genescreen Hybridization Transfer Membranes (Perkin Elmer, USA) by southern blotting, and the DNA was immobilized by ultraviolet cross-linking [49] . DNA replication intermediates present at either ChrIII or ChrVI were detected using unique chromosome-specific 32 P dCTP (6,000 Ci mmol −1 ; Perkin Elmer)-radiolabelled probes that were synthesized using the Rediprime II kit (GE Healthcare, Denmark). Stripping of membranes for subsequent reprobing was achieved by washing the membranes with a boiling solution of 0.1% SDS. Quantification of signals was performed using Image Quant analysis software (Molecular Dynamics, Sunnyvale, CA). Western blotting A modified version of the trichloroacetic acid (TCA) technique was used [50] . Cells were harvested by centrifugation, washed once and resuspended in 400 μl of 20% TCA. An equal volume of glass beads was added, and cells were disrupted using a FastPrep-24 instrument (MP Biomedicals, Denmark) for 4 × 20 s (full speed) cycles. Following disruption, 600 μl of 5% TCA was added and the samples were vortexed. The upper 600 μl was removed and this step was repeated, yielding 1.2 ml of supernatant. Following centrifugation at 5,700 r.p.m. for 5 min, the protein pellet was resuspended in Laemmli buffer (Bio-Rad, USA), and boiled for 3 min. Samples were again centrifuged, and the (soluble) protein extracts were separated by SDS-PAGE using 7% NuPAGE Tris-acetate gels (Invitrogen, UK). Rad53 was detected using a mouse monoclonal antibody (EL7; kindly provided by Dr Marco Foiani, IFOM, Milan, Italy) at a final dilution of 1:10. Horseradish peroxidase-linked secondary antibody was used at 1:4,000, and chemiluminescent detection was performed using an ECL kit (Thermo Scientific, Denmark). How to cite this article: Larsen, N. B. et al. The Escherichia coli Tus– Ter replication fork barrier causes site-specific DNA replication perturbation in yeast. Nat. Commun. 5:3574 doi: 10.1038/ncomms4574 (2014).